Bottom-up approach for the low-cost synthesis of graphene-alumina nanosheet interfaces using bimetallic alloys The production of high-quality graphene-oxide interfaces is normally achieved by graphene growth via chemical vapour deposition on a metallic surface, followed by transfer of the C layer onto the oxide, by atomic layer and physical vapour deposition of the oxide on graphene or by carbon deposition on top of oxide surfaces. These methods, however, come with a series of issues: they are complex, costly and can easily result in damage to the carbon network, with detrimental effects on the carrier mobility. Here we show that the growth of a graphene layer on a bimetallic Ni 3 Al alloy and its subsequent exposure to oxygen at 520 K result in the formation of a 1.5 nm thick alumina nanosheet underneath graphene. This new, simple and low-cost strategy based on the use of alloys opens a promising route to the direct synthesis of a wide range of interfaces formed by graphene and high-κ dielectrics. The coupling of graphene (Gr) with two-dimensional (2D) nanosheet dielectrics [1] , [2] , [3] , [4] is an important topic in contemporary materials science, due to its potential impact on a number of high-performance nanoelectronic applications [5] . In this respect, Al 2 O 3 films play a key role because of their employment as high-κ oxides in transistors and low-power chips, where the use of a high dielectric constant ( ε r =9; (ref. 6 ) increases the gate capacitance. Recent studies have reported a high mobility of exfoliated Gr in Al 2 O 3 /Gr interfaces synthesized using alumina nanoribbons (23,600 cm 2 V −1 s −1 ; (ref. 7 ) or ozone functionalization methods (19,000 cm 2 V −1 s −1 ; (ref. 8 ). However, the conventional methods so far used for producing Gr-alumina interfaces inevitably lead to a degradation of the electronic properties of Gr. Chemical vapour deposition (CVD) growth on transition metals [2] requires a transfer process involving the use of polymers, solvents, and etchants/water solutions which introduce contaminants or defects [9] , such as vacancies, grain boundaries and Gr multilayers. On the other hand, atomic layer deposition, used to directly synthesize oxide layers on top of Gr, typically requires a chemical modification of Gr to avoid wetting problems, and introduces impurities or causes C–C bond cleavages, leading to a significant degradation of the electron mobility. More recent strategies, based on Hf and Si deposition and subsequent oxidation, typically require expensive transition metal supports, such as Pt (ref. 10 ) and Ru (ref. 11 ). The intercalation of Al atoms to the Gr/Ni(111) interface and their subsequent oxidation has proven unsuccessful because of the surface segregation of the Al atoms, which results in the formation of an AlO x layer on top of graphene/Ni (ref. 12 ). Also the opposite approach, that is, the direct growth of graphene on top of oxide surfaces, has been tested. As an example, the CVD synthesis of graphene on sapphire [13] results in the formation of monolayer graphene with a charge carrier mobility >3,000 cm 2 V −1 s −1 , but requires very high temperatures (~1,800 K), which are not compatible with most of the Si CMOS processing. Zhou et al. [14] , on the other hand, were able to directly grow graphene on Co 3 O 4 (111) at lower temperature using molecular beam epitaxy from a solid carbon source, but the strong interaction they observed between the graphene layer and the substrate can largely contribute to electron scattering and reduce the charge mobility. By using molecular beam deposition above 970 K, Lippert et al. [15] achieved direct growth of graphene on alumina silicate, but they observed the coexistence of monolayers with bi- or multi-layer graphene flakes. It is therefore desirable to develop some alternative, scalable and economically affordable method for the transfer-free production of Gr-dielectric interfaces. Starting from a clean Ni 3 Al(111) surface ( Fig. 1a ), we here propose a novel approach for the direct synthesis of Gr-alumina interfaces, by growing Gr on the substrate by ethylene CVD ( Fig. 1b ) and subsequently oxidizing the metallic surface, in such a way to induce the formation of an alumina nanosheet ( Fig. 1c ). This method, based on the use of low-cost raw materials like NiAl, could be readily extended also to other alloys to produce high-κ dielectrics. 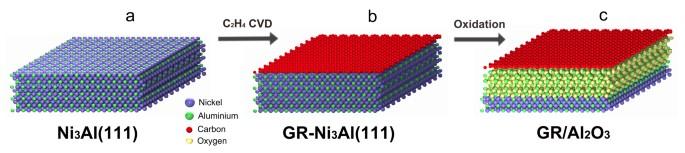Figure 1: Schematic outline of the present work. (a) The clean Ni3Al(111) surface, (b) Gr growth on Ni3Al(111) by means of high temperature ethylene CVD, and (c) oxidation of the Al atoms. Figure 1: Schematic outline of the present work. ( a ) The clean Ni 3 Al(111) surface, ( b ) Gr growth on Ni 3 Al(111) by means of high temperature ethylene CVD, and ( c ) oxidation of the Al atoms. Full size image Graphene synthesis on the Ni 3 Al(111) surface A graphene layer was first grown on Ni 3 Al(111) by ethylene CVD at 950 K, similar to the growth procedure used on Ni(111) (ref. 16 ) (see Methods). The first direct evidence of Gr formation on Ni 3 Al(111) comes from the C1s core level spectrum, presented in Fig. 2a . At low exposure we observe a peak at ~283.5 eV binding energy (BE), most probably due to C 2 H 4 fragments and carbides, while at larger carbon coverage a new component appears at higher BE (284.84 eV), attributed to Gr by comparison with Gr on Ni(111) (ref. 17 ). The integrated intensity of this peak shows a saturating behaviour, indicating a self-limiting growth process. In the final high-energy resolution C1s core level spectrum (measured at room temperature), the two components are separated by 410 meV (with the higher BE component at 284.84 eV) and exhibit a narrow line shape. 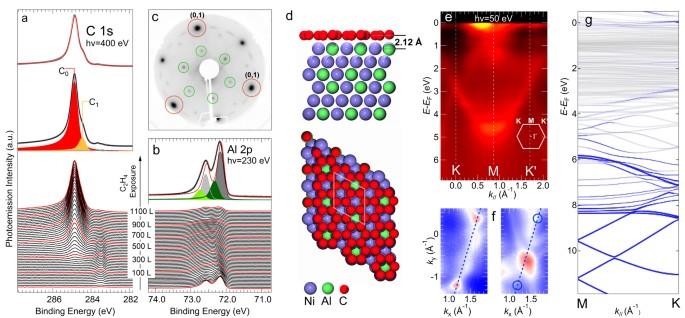Figure 2: Graphene on Ni3Al(111). (a) (bottom) C1s core level photoemission spectra acquired at different exposures during ethylene CVD at 950 K. (middle) High-resolution C1s core level spectrum measured at room temperature after Gr growth. The fit (black curve) and the C0(red) and C1(yellow) components are shown superimposed to the experimental data (grey circles). (top) Simulated C1s photoemission spectrum (red line) obtained from the DFT calculated binding energies for the top-fcc structure. (b) (bottom) Al2p core level photoemission spectra acquired at different exposures during ethylene uptake at 950 K. (top) High-resolution Al2p photoemission spectrum measured at room temperature after Gr growth. The fit (black curve) is shown superimposed to the experimental data (grey circles), along with the bulk (dark/light grey) and interface (dark/light green) components for the 2p3/2and 2p1/2sublevels. The Al2p spectrum obtained for the clean surface (red line) is plotted, after proper normalization, as a reference. (c) LEED pattern for the Gr/Ni3Al(111) system measured at 150 eV. (d) Top and side views for the top-fcc Gr/Ni3Al(111) structure. (e) ARPES measurement of the Gr/Ni3Al(111) energy band dispersion along the K–M–K′ direction in the reciprocal space and (f) constant energy surfaces at the Dirac point energy (left) and at the Fermi level (right). (g) DFT-calculated Gr energy band dispersion along the M–K direction for the top-fcc structure. The bands with a participation of 50% or more of carbon orbitals are highlight using blue lines. Figure 2: Graphene on Ni 3 Al(111). ( a ) (bottom) C1s core level photoemission spectra acquired at different exposures during ethylene CVD at 950 K. (middle) High-resolution C1s core level spectrum measured at room temperature after Gr growth. The fit (black curve) and the C 0 (red) and C 1 (yellow) components are shown superimposed to the experimental data (grey circles). (top) Simulated C1s photoemission spectrum (red line) obtained from the DFT calculated binding energies for the top-fcc structure. ( b ) (bottom) Al2p core level photoemission spectra acquired at different exposures during ethylene uptake at 950 K. (top) High-resolution Al2p photoemission spectrum measured at room temperature after Gr growth. The fit (black curve) is shown superimposed to the experimental data (grey circles), along with the bulk (dark/light grey) and interface (dark/light green) components for the 2p 3/2 and 2p 1/2 sublevels. The Al2p spectrum obtained for the clean surface (red line) is plotted, after proper normalization, as a reference. ( c ) LEED pattern for the Gr/Ni 3 Al(111) system measured at 150 eV. ( d ) Top and side views for the top-fcc Gr/Ni 3 Al(111) structure. ( e ) ARPES measurement of the Gr/Ni 3 Al(111) energy band dispersion along the K–M–K′ direction in the reciprocal space and ( f ) constant energy surfaces at the Dirac point energy (left) and at the Fermi level (right). ( g ) DFT-calculated Gr energy band dispersion along the M–K direction for the top-fcc structure. The bands with a participation of 50% or more of carbon orbitals are highlight using blue lines. Full size image The corresponding fast X-ray photoemission spectroscopy (XPS) measurements of the Al2p core level are clearly consistent with the formation of a Gr layer ( Fig. 2b ), which causes ~65% reduction of the Al2p integrated intensity. The high-resolution Al2p spectrum of Gr-covered Ni 3 Al, compared with that of the clean sample (shown superimposed in Fig. 2b ), shows an additional spin-orbit doublet (green components), shifted by +160 meV, which is assigned to the interacting Al atoms at the metal-Gr interface. The low energy electron diffraction (LEED) pattern of the Gr/Ni 3 Al(111) interface, reported in Fig. 2c , shows the same (2 × 2) hexagonal periodicity observed for the clean substrate [18] (green circles in Fig. 2c ), indicating that the first bimetallic layer, which has a lattice mismatch of only 2.4% with respect to Gr, has not undergone any reconstruction or structural modification. Some differences from the clean case are detectable, in particular, a very weak ring-shaped modulation revealing the presence of residual differently oriented Gr domains, as previously reported for Ni(111) (ref. 19 ). To get a more detailed insight into the structure and properties of the Gr/Ni 3 Al system, we performed Density Functional Theory (DFT) calculations for six possible high-symmetry configurations obtained by imposing the constraint that Gr forms a (2 × 2) superstructure on Ni 3 Al(111) (see Supplementary Information ). In particular, we focused our attention on the top-fcc, top-hcp, fcc-hcp, b-top, b-fcc and b-hcp structures, each of which is characterized by a different arrangement of the carbon atoms relative to the Ni substrate atoms (see Supplementary Fig. 1 ). We found that the minimum energy configuration is the b-top, followed by the top-fcc ( Fig. 2d ), separated by only 60 meV, similarly to what was obtained in the DFT calculations for Gr on Ni(111) (ref. 20 ); see Supplementary Table 1 ). The b-fcc and b-hcp are not stable and relax into a top-fcc and top-hcp structure, respectively. Finally, the top-hcp and fcc-hcp configurations turn out to be the least stable, with a significantly higher energy. Angle-resolved photoemission (ARPES) measurements ( Fig. 2e,f ) show the disruption of the Dirac cone, with the whole π-band of the Gr layer shifted to higher BE with respect to free-standing Gr. This is similar to what has been reported for Gr on Ni(111) (ref. 16 ) and results from the strong hybridization between the Gr and metal 3d valence band states. In particular the bottom of the band, at the M point, is ~4.7 eV below the Fermi level, while the Dirac point is found at ~2.7 eV. The high density of states at the Fermi level ( E F ), instead, is mainly due to the Ni d-band of the alloy substrate. The calculated band structure for the top-fcc Gr-Ni 3 Al(111) geometry ( Fig. 2g ) shows an excellent agreement with the experimental data, supporting the hypothesis that the observed structure is predominantly top-fcc. To further understand which of the two minimum energy structures corresponds to the experimentally observed one, we calculated the C1s core electron binding energies for all the non-equivalent carbon atoms (see Methods, Supplementary Fig. 2 and Supplementary Table 2 ). By comparing the simulated photoemission spectrum for the two cases, we found a better agreement for the top-fcc structure, as reported in the top panel of Fig. 2a (red line). However, the coexistence of the two phases cannot be excluded. Finally, for the top-fcc structure, the calculated mean distance between the Gr layer and the substrate is 2.12 Å, similar to the Gr-Ni(111) system [20] . The graphene-alumina nanosheet interface After Gr growth, the Gr–alloy interface was exposed to a high flux of molecular oxygen (pressure=3 × 10 −3 torr) at 520 K. Following this procedure, it is possible to intercalate oxygen underneath the Gr layer and to selectively oxidize only the Al atoms at the metal interface. In fact, the intercalation of noble or light atoms has already proven to be an effective method to create an interface nanosheet between Gr and the substrate [21] , [22] , [23] , [24] . 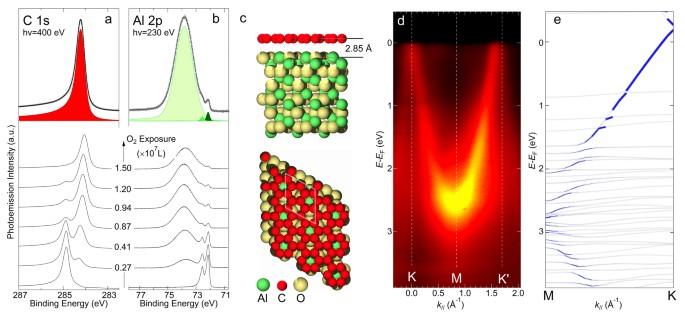Figure 3: Oxygen intercalation underneath graphene. (a,b) (bottom) C1s and Al2p photoemission spectra acquired at different O2exposure. (top) C1s and Al2p high-resolution spectra acquired after the formation of a thick alumina nanosheet underneath Gr, the fit components are shown superimposed to the experimental data. (c) Top and side views of the simulated Gr/Al2O3structure. (d) ARPES measurement of the Gr/Al2O3electronic band structure along the K–M–K′ direction. (e) DFT calculated energy band dispersion for the Gr/Al2O3system. Figure 3a,b shows a set of high-resolution photoemission spectra acquired after different oxygen exposures, for the C1s and Al2p levels, respectively. Looking at the C1s spectrum, we observe the appearance of a new component at lower BE with respect to the previously described Gr peak. From a comparison of our data with previous literature [11] , [25] , we ascribe this new component to regions of Gr sitting on an oxide substrate. As the oxygen dose increases, this new peak grows in intensity at the expense of the previous one, indicating that oxide layer formation proceeds through the nucleation and progressive expansion of islands. Finally, above 10 7 l of oxygen exposure (1 l=1 × 10 −6 torr s), the signal associated with Gr/NiAl basically disappears from the spectrum. After the carbon layer has been completely decoupled from the substrate, the C1s spectrum shows a single, narrow component centred at 284.2 eV, which, notably, is shifted by ~590 meV to lower BE with respect to the higher BE C1s components (C 0 ) of Gr/Ni 3 Al(111). It is important to note that, during intercalation, the total C1s intensity decreases by <5%, indicating that the overall integrity of the carbon network is preserved. The C1s spectral shift to lower BE, which is an indication of charge transfer from graphene to the electronegative oxygen atoms, resulting in hole-doped graphene, cannot be uniquely attributed to initial-state effects, but can also receive a contribution, although smaller, from final-state mechanisms, that is, core hole screening. Similar effects have also been reported by Katsiev et al. [26] for oxygen intercalation at the Gr/Ru(0001) interface. Figure 3: Oxygen intercalation underneath graphene. ( a , b ) (bottom) C1s and Al2p photoemission spectra acquired at different O 2 exposure. (top) C1s and Al2p high-resolution spectra acquired after the formation of a thick alumina nanosheet underneath Gr, the fit components are shown superimposed to the experimental data. ( c ) Top and side views of the simulated Gr/Al 2 O 3 structure. ( d ) ARPES measurement of the Gr/Al 2 O 3 electronic band structure along the K–M–K′ direction. ( e ) DFT calculated energy band dispersion for the Gr/Al 2 O 3 system. Full size image The selective oxidation of the Al atoms in the first few layers was monitored by following the evolution of the Al2p core level spectra acquired at increasing oxygen exposure ( Fig. 2b ). As oxygen intercalation proceeds, we observe the growth of a broad peak, centred at about 73.8 eV, in the same BE region as the signal that typically accompanies the formation of an alumina film on NiAl alloys [27] . On the other hand, as it is clear from the evolution of the Ni2p 3/2 spectra, the Ni atoms are almost unaffected by the oxidation process. This finding can be explained in terms of a thermally promoted surface segregation of the Al atoms, resulting in a Ni-depleted first layer. Since the oxide layer is mainly formed by alumina, we were able to estimate the oxide layer thickness from the intensity decrease of the Ni2p 3/2 signal. The estimated mean thickness of the alumina layer, taking into account the inelastic photoelectron mean free path, is ~1.5±0.2 nm. The BE difference between the C1s and Al2p core levels measured in our work (Δ E =210.2 eV) is very similar to the value found in the case of Gr grown on sapphire (Δ E =210.3 eV; ref. 13 ), where the Al2p has been used for calibration, thus indicating the close similarities between the two systems. It is important to underline the absence of any interfacial buffer layer between Gr and alumina, which would give rise to a feature at 281.5 eV (the BE corresponding to the Al–C bonds) and 282.5 eV (Al–O–C bond) [28] , [29] and also to C–O bonds characteristic of epoxy, ethers, quinones and lactones, which typically show up in the C1s spectrum at binding energies>284.2 eV (ref. 22 ). In addition, we can safely rule out the formation of a high density of Gr defects such as single- and double-vacancies or Stone–Wales defects. Based on DFT calculations performed on both Highly Oriented Pyrolitic Graphite [30] and Gr (ref. 31 ), the presence of this kind of defects in a concentration >1% would clearly show up in our high-resolution core level spectra in the form of lower BE components. The DFT-calculated structure for a Gr layer on the Al 2 O 3 (0001) α-phase ( Fig. 3c ), which approximately reproduces the experimentally obtained thick alumina layer (see methods), shows a distance of 2.85 Å between Gr and the oxide substrate. The ARPES measurements, reported in Fig. 3d , show that the Dirac cone in the vicinity of the Fermi energy is fully restored, thus confirming that Gr lies on top of a thick oxide layer, which decouples it from the metallic alloy. In particular, the bottom of the π band at the M point shifts by about 2 eV, with the Dirac point lying above the Fermi energy. Moreover, close to the K and K′ points, the energy dispersion becomes linear, as expected for quasi-free-standing Gr. From a linear fit of the dispersion curve close to the K point, we estimated that the group velocity of the charge carriers (d E (k)/dk) is~8 × 10 5 m s −1 (~1/370 of the speed of light), in good agreement with the theoretically predicted value for free-standing Gr. From a linear extrapolation, we estimated that the Dirac point is 200±40 meV above E F , thus indicating an oxide-induced p-doping of the Gr layer. The DFT calculated electronic dispersion shows an excellent agreement with the experimental data. In particular, the bottom of the π-band and the region near the Dirac point are well-reproduced ( Fig. 3e ). The calculated band energy value at the K point lies 220 meV below E F , consistent with the experimental value. Graphene quality after the oxidation process To assess the quality of the Gr layer after oxidation, we compared the LEED patterns, acquired at the same electron energy ( E =71 eV, where the first order diffraction spots of Gr are particularly intense), of the following structures: (a) clean Ni 3 Al(111), (b) Gr/Ni 3 Al(111) and (c) Gr/Al 2 O 3 (see Fig. 4 ). The transition from a threefold (a) to a sixfold (b) symmetry in the circular line profile is consistent with the formation of a single-Gr layer on top of Ni 3 Al(111). Most importantly, the periodicity and symmetry are preserved after alumina growth underneath Gr/Ni 3 Al, although with an increased background due to the small corrugation of the graphene layer and to scattering from the disordered alumina substrate (whose (2 × 2) periodicity disappears). The half width at half maximum (HWHM) of the diffraction spots remains almost unchanged from the Gr/Ni 3 Al to the Gr/Al 2 O 3 structure, thus suggesting that the long-range structural order is largely preserved upon oxidation. The small increase (only 9%) in the HWHM of the spots is interpreted as due to the corrugation of the alumina layer (see also description of the low energy electron microscopy (LEEM) experiments). In this respect, it is important to stress that the roughness of epitaxial Gr on SiO 2 is always found to be larger than that of free-standing Gr, because of the energetic cost of the elastic deformations, which prevent the Gr layer from exactly conforming to the substrate morphology [32] , [33] . 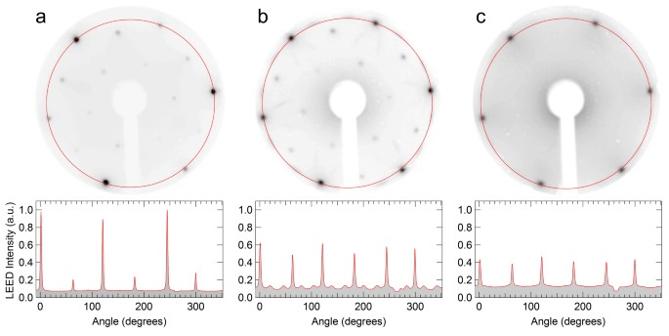Figure 4: LEED patterns of the different phases. Low energy electron diffraction patterns of the (a) clean Ni3Al(111), (b) Gr/Ni3Al(111) and (c) Gr/Al2O3structures acquired at the same electron energy (71 eV). The bottom panel represents the corresponding circular diffraction profiles, as shown in the top images (red circles). Figure 4: LEED patterns of the different phases. Low energy electron diffraction patterns of the ( a ) clean Ni 3 Al(111), ( b ) Gr/Ni 3 Al(111) and ( c ) Gr/Al 2 O 3 structures acquired at the same electron energy (71 eV). The bottom panel represents the corresponding circular diffraction profiles, as shown in the top images (red circles). Full size image To shed further light on the structural and morphological quality of the Gr layer on the nanoscale, we employed LEEM and microprobe-diffraction (μ-LEED). Our experiments showed that Gr on Al 2 O 3 extends continuously across the sample, nicely confirming that Gr is not etched upon substrate oxidation. To assess the film rotational structure, we employed the dark-field (df) imaging mode, utilizing one of graphene’s first order diffraction beams to map the lateral size of single crystal domains. As can be seen in Fig. 5a,d , the film is composed by rather large tiles, each one extending for several microns. A few nanometer-size dark features are observed within some of them, suggesting that the structure of the oxidized substrate may be locally inhomogeneous. As can be seen in Fig. 5b , our diffraction experiments show that the majority of the Gr crystals are epitaxial, that is, they are exactly in registry with the substrate. Similar to the case of Gr on Ni 3 Al(111) ( Fig. 4b ), rotated crystals are also observed (see Fig. 5d ), with the Gr unit vectors aligned at ~±16° with respect to the main substrate directions. These flakes are, on an average, smaller than the epitaxial ones and exhibit a slightly lower rotational coherence across the sample. 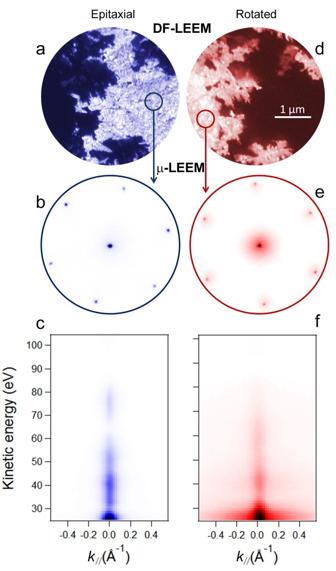Figure 5: LEEM and microprobe-LEED experiments. df-LEEM image of (a) an epitaxial and (d) a rotated Gr flake (Start voltage: 40 eV). The two images, which were obtained using the corresponding first order diffraction beams, map the lateral extent of two distinct Gr single-crystals within the same microscopic region of the sample. (b,e) μ-LEED pattern from the same two single-crystals, as measured by probing an area of diameter 500 nm. Electron energy is 50 eV. Waterfall plot of a cross-section though the zero-order diffraction spot of (c) an epitaxial and (f) a rotated Gr flake as a function of the electron energy. Figure 5: LEEM and microprobe-LEED experiments. df-LEEM image of ( a ) an epitaxial and ( d ) a rotated Gr flake (Start voltage: 40 eV). The two images, which were obtained using the corresponding first order diffraction beams, map the lateral extent of two distinct Gr single-crystals within the same microscopic region of the sample. ( b , e ) μ-LEED pattern from the same two single-crystals, as measured by probing an area of diameter 500 nm. Electron energy is 50 eV. Waterfall plot of a cross-section though the zero-order diffraction spot of ( c ) an epitaxial and ( f ) a rotated Gr flake as a function of the electron energy. Full size image The crystal quality of epitaxial and rotated flakes exhibits similar characteristics, as is revealed by careful analysis of the μ-LEED pattern. Epitaxial Gr displays a purely Gaussian line-shaped profile, with HWHM<0.06 Å −1 . This value is much smaller than those reported for both SiO 2 -supported and suspended exfoliated single-layer Gr (ref. 34 ), the former being the reference material used in graphene prototypical devices and is indicative of excellent crystal quality. In rotated domains, the diffraction beam-line profile is predominantly Gaussian, with HWHM<0.08 Å −1 , indicating similar crystal quality to that observed in epitaxial Gr flakes. As can be seen in Fig. 5c,f , where line profiles measured across the zero-order diffraction beam are reported for epitaxial and rotated flakes respectively, no significant peak broadening can be observed as a function of the increasing electron energy, from which we conclude that no significant corrugation occurs at length scales <20 nm (ref. 34 ). To understand the effect of the Gr layer on the oxidized substrate in comparison to the clean surface, we performed a series of oxidation experiments on bare Ni 3 Al(111). 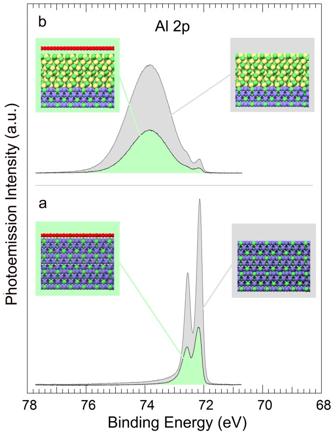Figure 6: Alumina layer properties of clean and graphene covered samples. Al 2p photoemission spectra acquired in similar condition for the clean (grey) and Gr-covered (green) sample: (a) clean substrate and (b) after formation of an alumina nanosheet. Figure 6 shows a set of photoemission spectra of the clean and Gr-covered sample measured under similar oxygen coverage conditions. The Al2p spectra measured before and after Gr growth are reported in Fig. 6a . The clean Ni 3 Al crystal was first exposed to an O 2 pressure of 4 × 10 −7 torr at 520 K, approximately up to the same coverage reached in the oxygen intercalation experiment ( Fig. 4 ). After oxidation, the Al2p spectrum is comparable to the one obtained in the presence of Gr, apart from an intensity enhancement due to the absence of the carbon layer. In particular, both spectra show a broad peak centred at the same BE (73.8 eV), while a residual signal arising from the metallic Al atoms is still present. This suggests that oxygen intercalation on the Gr-covered sample at 520 K leads to the formation of an oxide layer with the same composition as the one obtained upon oxidation of the clean substrate. Notably, the effect of Gr on the Al2p signal reduction amounts to 65% in both cases. In conclusion, our findings suggest that the presence of the Gr layer plays a minor role in the oxide layer structure. Figure 6: Alumina layer properties of clean and graphene covered samples. Al 2p photoemission spectra acquired in similar condition for the clean (grey) and Gr-covered (green) sample: ( a ) clean substrate and ( b ) after formation of an alumina nanosheet. Full size image Besides its simplicity, the method we have developed offers the advantage of using low-cost raw materials which can be easily processed by conventional metal powder technology. Our method could be used also with other Al-based bimetallic alloys (CuAl 2 , CoAl, FeAl, Fe 3 Al) capable of breaking the C–H bonds in hydrocarbon molecules and of selectively oxidizing the Al atoms. The availability of a large range of low-cost bimetallic compounds (NiZr, NiTi and so on) can open new avenues for Gr-integrated materials with higher dielectric constant (ZrO 2 ε r =25, TiO 2 ε r =30 (anatase)–100 (rutile) and so on) than conventional SiO 2 ( ε r =3.9). The coupling of Gr with oxide nanosheets could also be exploited in spin-filtering materials, to remove the spin-scattering effects arising when the Gr layer is directly supported on transition metals. The thickness of the so-produced oxide layer is comparable to the values used in the latest high-efficiency spin transport devices. Finally, other oxide layers could be deposited, by means of well-established methods, on top of the Gr–oxide interface, in such a way to build oxide–Gr–oxide sandwiched heterostructures, which represents a fundamental architecture in most new generation electronic devices. Sample preparation The Ni 3 Al(111) single crystal used in this work was polished before the experiment, then cleaned in ultra-high vacuum (UHV) conditions by repeated cycles of 2 keV Ar + sputtering and annealing to 1,170 K. This procedure ensured a high-quality surface, as judged by LEED and XPS. The measurements reported in this work were also performed in UHV conditions, with a background pressure of the order of 1 × 10 −10 torr. Procedure for graphene growth The graphene layer was grown on Ni 3 Al(111) by ethylene (C 2 H 4 ) CVD at 950 K, using a maximum partial pressure of 1.5 × 10 −6 mbar, up to a total C 2 H 4 exposure of about 10 3 l. These parameters were chosen to reduce the probability of carbon dissolution into the bulk and, at the same time, obtain a high-quality graphene layer. In particular, a high pressure was needed to ensure a fast formation of nucleation seeds, while a high temperature was selected to enhance the carbon surface mobility, and hence to promote their surface diffusion and the subsequent formation of an ordered graphene layer. Higher temperatures were not used in the present experiment because of the thermally enhanced carbon bulk solubility. X-ray photoelectron spectroscopy The high-energy resolution XPS and fast XPS experiments were carried out at the SuperESCA undulator beamline of the Elettra synchrotron radiation facility (Basovizza, Italy). The photoemitted electrons were collected and analyzed by a state-of-the-art SPECS PHOIBOS 150 hemispherical analyzer equipped with a delay line detector developed at Elettra. The C1s, Al2p, Ni2p 3/2 and O1s spectra with their corresponding Fermi levels were acquired with a photon energy of 400 eV, 230 eV, 950 eV and 650 eV, respectively. All the spectra were measured in the normal emission geometry. A linear background was always subtracted from the core level signal, except for the Ni2p 3/2 spectra, for which a Shirley-type background was instead used. The spectra were then offset by the corresponding Fermi energies and fitted to a multipeak Doniach–Šunjić function convoluted with a Gaussian. Angle-resolved photoemission spectroscopy The ARPES measurements were performed at the SGM3 undulator beamline of the ASTRID storage ring in Aarhus (Denmark). The 2D detector, consisting of a phosphor screen coupled with a high-resolution CCD camera, combined with a PHOIBOS 150 hemispherical analyzer, yields an angular resolution better than 0.15° and an energy resolution of the order of 10 meV. The angle-resolved spectra were acquired with a photon energy of 50 eV. Low energy electron diffraction The LEED experiments were performed in the UHV chamber of the Surface Science Laboratory at Elettra-Sincrotrone Trieste using a VG rear-view electron optical system. Low energy electron microscopy The LEEM and microprobe-LEED data were collected with the spectroscopic photoemission and low energy electron microscope (SPELEEM III, Elmitec GmbH) at the Nanospectroscopy beamline of Elettra. In the microscopy mode, elastically backscattered electrons are used to image the specimen surface with a spatial resolution of up to 10 nm. By imaging the objective lens backfocal plane, the microscope allows also operation in the diffraction mode. LEED patterns from selected microscopic surface regions are obtained by restricting the size of the illuminating electron beam by means of an aperture. The smallest aperture allows probing an area of diameter 500 nm. Gr on the oxidized Ni 3 Al sample was prepared ex situ and transferred through air to the SPELEEM chamber. Prior to the LEEM measurements the sample was mildly heated up to about 400 K. Density functional theory calculations The DFT [35] , [36] calculations were performed with the VASP code [37] . We employed a plane-wave basis set including all plane waves up to a kinetic energy of 400 eV, and the core electrons were treated with the Projector Augmented Wave method [38] as implemented in VASP (ref. 39 ). Spin-polarized calculations were performed with several different functionals, among which we included the LDA, PBE [40] , Grimme [41] and Dion et al. [42] functionals. A 2 × 2 slab of Ni 3 Al(111) containing 18 Ni atoms and 6 Al atoms (a total of six layers) was employed to simulate the surface, with a vacuum region above the slab of ~16.5 Å. The three bottom layers were frozen in their atomic bulk positions, while the remaining layers were allowed to relax. The structural relaxation was performed using the conjugate gradients algorithm. Once the slab geometry had been optimized, an 8-C-atom Gr slab was placed on top of it in various configurations, as discussed in the text, and the resulting structures were relaxed once again. The same procedure was used to simulate Gr on the α-phase of Al 2 O 3 (0001). In this case the slab consisted of 12 Al and 18 O atoms. Apart from this, the calculations were carried out in the same way as for the Ni 3 Al-Gr case. Our relaxation calculations with the various exchange-correlation functionals revealed that both the PBE [40] and Dion et al. [42] functionals find no favourable interaction between Gr and the Ni 3 Al substrate, in open contradiction with the experimental results. In contrast, the Local Density Approximation (LDA) and Grimme [41] functionals provide very consistent results, indicating that the bridge-top is the most favourable structure, closely followed by the top-fcc arrangement, which was predicted to be 0.06 eV less stable (meaning a difference of <0.01 eV per C atom). All subsequent calculations were thus performed with the LDA functional. The core electron binding energies were calculated in the final-state approximation. A standard calculation was first performed on the fully relaxed system, then an electron from the selected core level of the atom under consideration was excited into the lowest conduction state, and the electronic structure re-calculated at fixed atomic positions. The difference between these two energies yields an estimate of the initial core level BE. Calculated geometries of graphene/Ni 3 Al(111) Six non-equivalent geometries that were investigated for the graphene/Ni 3 Al(111) system (see Supplementary Fig. 1 ). These configurations were chosen due to their symmetric properties and can be obtained from one another by a rigid shift of the graphene layer along a C–C bond direction. They are named after the two adsorption sites occupied by the two non-equivalent carbon atoms in the graphene network, with respect to the substrate. In Supplementary Table 1 we also report their calculated energies as obtained by DFT calculations of cells containing an 8-C-atom graphene layer. C1s core level fitting procedure The experimental C1s spectrum was fitted to a sum of Doniach–Šunjić functions. Since DFT predicts the relative BE shifts among components, rather than the absolute values, the experimental and theoretical BE scales were originally offset. We corrected for this offset by including it as a free fitting parameter in our procedure, while holding the relative shifts fixed to their theoretically calculated values. The Lorentzian and Gaussian widths, as well as the asymmetry parameter, were constrained to be the same for all peaks. This is equivalent to assuming that: the core electronic states corresponding to each atomic configuration have the same finite lifetime (resulting in an equal Lorentzian broadening); all the core level components are affected to the same extent by thermal phonon broadening, experimental and inhomogeneous broadening (which are reflected in their Gaussian FWHM); the chance of an electron–hole pair excitation event is the same for all core level components. Our choice was required to rationalize the fitting procedure and reduce the number of degrees of freedom. In addition, we constrained also the photoemission intensity to be the same value for all components. The analysis was carried out in two steps: we first tested the agreement between our experimental data and the DFT-simulated C1s spectrum for the b-top structure, then we repeated the same procedure for the top-fcc configuration. As reported in Supplementary Table 2 , in the b-top structure, C atoms are found in three non-equivalent configurations, yielding six different core level BEs: top Al, where a C atom is directly above a surface Al atom, and two bridge configurations in which a C–C bond lies directly on top of a Ni atom, which can be either at the centre of the cell (b-Ni c ) or halfway along a lattice vector (b-Ni s ). Since the population of C atoms in b-Ni s configuration is twice as large as the other two, two pairs of C atoms within the simulation cell are degenerate in BE. For this reason, we used a six peak fitting function where two components are twice as intense as the other four. The agreement between experimental data and DFT simulations for the b-top structure is very good, as is clear from Supplementary Fig. 2 (left). As the second step, we repeated the above analysis for the top-fcc structure. In this case, as seen in Supplementary Table 2 , four non-equivalent populations of C atoms can be identified within the simulation cell, each of which is twofold degenerate: more specifically, we have two configurations with a C atom at a threefold fcc hollow site (fcc-Ni 3 and fcc-Ni 2 Al), and two configurations with a C atom on top of a Ni (top-Ni) or an Al atom (top Al), respectively. For this reason, for our analysis it was enough to use a four-peak fitting function. This structure, as judged from a χ 2 -analysis, yields an overall better agreement with the experimental photoemission data, especially for the lower BE part ( Supplementary Fig. 2 (right)). How to cite this article: Omiciuolo, L. et al. Bottom-up approach for the low-cost synthesis of graphene-alumina nanosheet interfaces using bimetallic alloys. Nat. Commun. 5:5062 doi: 10.1038/ncomms6062 (2014).